Adhesive water networks facilitate binding of protein interfaces Water structure has an essential role in biological assembly. Hydrophobic dewetting has been documented as a general mechanism for the assembly of hydrophobic surfaces; however, the association mechanism of hydrophilic interfaces remains mysterious and cannot be explained by simple continuum water models that ignore the solvent structure. Here we study the association of two hydrophilic proteins using unbiased extensive molecular dynamics simulations that reproducibly recovered the native bound complex. The water in the interfacial gap forms an adhesive hydrogen-bond network between the interfaces stabilizing early intermediates before native contacts are formed. Furthermore, the interfacial gap solvent showed a reduced dielectric shielding up to distances of few nanometres during the diffusive phase. The interfacial gap solvent generates an anisotropic dielectric shielding with a strongly preferred directionality for the electrostatic interactions along the association direction. Although hydrophilic protein interfaces are often involved in the formation of protein complexes, the mechanism that describes how such surfaces assemble is not well characterized. Most of the previous computational studies on protein folding and association have dealt with hydrophobic interfaces [1] , [2] , [3] , [4] , [5] . In that case, hydrophobic dewetting has been shown to be an essential driving force in biology [3] , [4] , [5] , [6] . Recently, several studies have pointed out that dewetting is rare [7] , [8] , [9] , [10] because a few polar residues can prevent the occurrence of dewetting [8] , [9] . Taking into account the fact that on average ∼ 70% of the interfacial residues of protein complexes are hydrophilic, including ∼ 37% charged residues [11] , hydrophilic interfaces are clearly of larger importance for assembly. The association of hydrophilic surfaces is traditionally thought to result from the direct electrostatic interactions between the binding partners. A recent neutron diffraction study showed an example in which the association between some small peptides was dominated by charge–charge rather than hydrophobic interactions [12] . However, the simple picture of coulombic interactions screened by a continuum solvent is not able to fully explain the complicated nature of hydrophilic interactions. In particular, the continuum description of water ignores the important role that the structure of the water network has for the interaction between water and solute molecules. Such a role has been well documented for the case of hydrophobic interactions in which it also showed an interesting size dependence [3] , [4] . In contrast, the mechanistic role of the water structure in hydrophilic interactions is poorly understood especially for large hydrophiles, such as proteins. Here, using extensive molecular dynamics (MD) simulations with explicit water representation, we aim to find the basis of atomistic mechanisms during association of hydrophilic interfaces. Our simulations for the binding process of Barnase–Barstar reproducibly recover the native bound state of the complex and thus provide atomistic insight into the mechanism of binding. The simulations showed that water in the interfacial gap forms an adhesive hydrogen-bond network between the hydrophilic protein interfaces. This network has an important role in stabilizing the early intermediate states before native contacts are formed. The transformation from these intermediates to the stereospecific complex is then accompanied by maximization of the interfacial water mediation. Furthermore, water structure has an important long-range role during the diffusive phase in reducing the dielectric shielding of water. The dielectric constant in the gap between the proteins is strongly reduced up to distances of a few nanometres. Interestingly, the dielectric properties of the water in the interfacial gap are strongly anisotropic with a preferred directionality for the electrostatic interactions along the direction perpendicular to the interfaces. Therefore, the water solvent between the two proteins makes an important contribution to the electrostatic funnelling of the binding free energy surface for the binding process. Simulations of the binding process We studied the protein–protein complex of Barnase–Barstar, which binds through a clearly hydrophilic binding interface (see Supplementary Fig. S1 ). The reason behind choosing this system is the availability of a wealth of experimental and computational data for the association of this model complex. Although it is well known that electrostatic interactions are responsible for the tight and fast binding, [13] , [14] , [15] , [16] , [17] , [18] , [19] as well as for stabilizing the intermediate complexes [14] , the atomistic mechanism of binding, especially the dynamic transformation from the encounter complexes to the stereospecific complex and the role of solvent is still not understood. Thus, we present here results from a series of atomistic MD simulations with explicit solvent representation starting from various unbound conformations. These were generated by displacing the two proteins from the bound state in the crystal complex [13] to an interfacial distance of 1.2–2.3 nm (see Supplementary Fig. S2 ). The total simulation time was 1.64 μs. Five simulations out of nine resulted in bound conformations very close to the crystal complex within the simulation time (see Supplementary Table S1 ). Three of these simulations had a minimum root mean square deviation (RMSD) <0.13 nm from the backbone coordinates of the crystal complex ( Supplementary Fig. S3 ) so that they are practically indistinguishable from the native bound conformation. The binding process took place on timescales of hundreds of nanoseconds and consisted of three different phases, as we observed in a previous work [5] . Diffusion led to intermediate transient encounter complexes [20] , of which some proceeded very close to the stereospecific complex. The diffusive phase only lasted a very short time with the first contacts forming within 2 ns. After the short diffusive phase, intermediate complexes were formed with a spatial orientation close to the stereospecific complex (RMSD <0.5 nm). The early intermediate complexes only had a few native crystal contacts formed ( Fig. 1a,b ). This is in agreement with double mutant cycle analysis for this complex, according to which the transition state for association occurs before most interactions are established [14] . The main conformational changes during the transition to intermediate states are rearrangements of the side chains and of the interfacial water molecules. The conformational changes towards the final stereospecific complex took place on a timescale of hundreds of nanoseconds; most of the native contacts were formed within 50–200 ns ( Fig. 1a,b ). 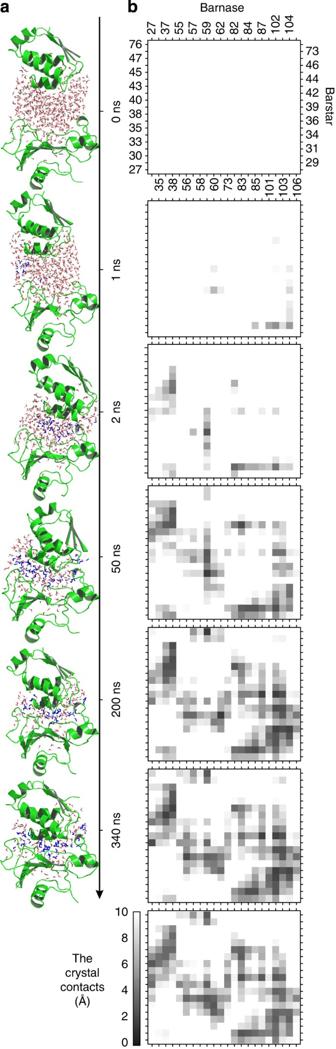Figure 1: Conformational snapshots along the binding pathway. (a) Snapshots at different simulation times showing the transformation from the starting structure to the final complex through binding intermediates (from sim1). Only solvent molecules in the interfacial gap are shown. The water molecules that belong to the hydrogen-bonded hydration shells of both proteins are coloured blue. The graphics were generated using PYMOL55. A movie for the binding process is available in theSupplementary Movie. (b) Contact maps between Barnase–Barstar for different snapshots in comparison with the native crystal contacts. The minimum distance between heavy atoms is computed for each pair of the interfaces. Figure 1: Conformational snapshots along the binding pathway. ( a ) Snapshots at different simulation times showing the transformation from the starting structure to the final complex through binding intermediates (from sim1). Only solvent molecules in the interfacial gap are shown. The water molecules that belong to the hydrogen-bonded hydration shells of both proteins are coloured blue. The graphics were generated using PYMOL [55] . A movie for the binding process is available in the Supplementary Movie . ( b ) Contact maps between Barnase–Barstar for different snapshots in comparison with the native crystal contacts. The minimum distance between heavy atoms is computed for each pair of the interfaces. Full size image Hydrogen-bonded network between the proteins During the simulations, the most significant property of the intermediate complexes is the highly solvated state of the interfaces. A total of 60–80 water molecules were constantly present in the interfacial gap (within 0.5 nm of both interfaces) showing that the interfaces did not undergo dehydration but rather remained highly hydrated even in the final stereospecific complex. To further characterize the properties of these interfacial waters, we computed the water density in the interfacial gap (see Methods ) and its distance dependence as before [5] ( Fig. 2a ). In comparison to the previous study on hydrophobic interfaces, the interfacial water density did not show any dewetting here even at close separation distances. On the contrary, the water density was never lower than that in bulk and was even a bit higher at closer distance ( Fig. 2a ). Moreover, the fluctuations of water density for the complex were comparable to those for the individual proteins and even smaller at close distances ( Supplementary Fig. S4 ). This means that the hydration shells do not become softer, as was found for hydrophobic interfaces [21] , [22] . One possible role for the solvated nature of encounter intermediates is to ease the conformational changes for reaching the specific complex concomitant with the supposed role of water as a lubricant for the fast conformational changes [23] . 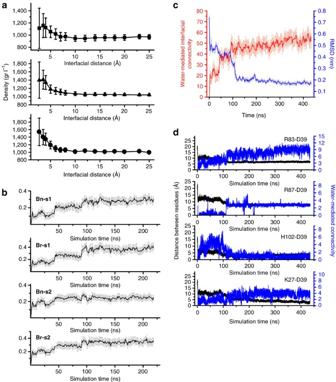Figure 2: Structural properties of the water in the interfacial gap. (a) Water density in the interfacial gap for different interfacial distances for the complex (squares) and around the individual proteins (Barnase (triangles) and Barstar (circles)). The water density was averaged over the last 1.7 ns for each 2-ns position-restrained molecular dynamics simulation. The error bars represent the standard deviation when taking the average. The gap was defined as in the calculation of the electric susceptibility (seeMethods). The gaps for the independent chains were defined by superposition of the corresponding part from the complex simulation to all snapshots of the independent protein–water system. (b) Development of water bridges between the interfaces (from sim1). The hydrogen-bonded water shells were defined as the water molecules that are directly bound to the interfaces with hydrogen bonds (the first shell s1) and the water molecules bound to s1 (the second shell s2). A water molecule in a shell was considered shared if it belonged to the s1 or s2 shells of both proteins. The shared fraction with the other chain was computed for each shell for both Barnase (Bn) and Barstar (Br). The values were averaged over time intervals of 1 ns and the standard deviations are presented as the error bars. (c) Water-mediated interfacial connectivity (red line from sim1) and the root mean square deviation root mean square deviation (RMSD; blue line). The values were averaged over intervals of 2 ns. The error bars represent the standard deviations. The water-mediated interfacial connectivity increased throughout the binding pathway. It shows a clear anti-correlation with the RMSD of −0.75. (d) Examples of the pairwise water-mediated connectivity. Four different pairs are shown with known high cooperative energy. The water-mediated connectivity is formed before specific contacts are established. The connectivity values were averaged over intervals of 1 ns. Figure 2: Structural properties of the water in the interfacial gap. ( a ) Water density in the interfacial gap for different interfacial distances for the complex (squares) and around the individual proteins (Barnase (triangles) and Barstar (circles)). The water density was averaged over the last 1.7 ns for each 2-ns position-restrained molecular dynamics simulation. The error bars represent the standard deviation when taking the average. The gap was defined as in the calculation of the electric susceptibility (see Methods ). The gaps for the independent chains were defined by superposition of the corresponding part from the complex simulation to all snapshots of the independent protein–water system. ( b ) Development of water bridges between the interfaces (from sim1). The hydrogen-bonded water shells were defined as the water molecules that are directly bound to the interfaces with hydrogen bonds (the first shell s1) and the water molecules bound to s1 (the second shell s2). A water molecule in a shell was considered shared if it belonged to the s1 or s2 shells of both proteins. The shared fraction with the other chain was computed for each shell for both Barnase (Bn) and Barstar (Br). The values were averaged over time intervals of 1 ns and the standard deviations are presented as the error bars. ( c ) Water-mediated interfacial connectivity (red line from sim1) and the root mean square deviation root mean square deviation (RMSD; blue line). The values were averaged over intervals of 2 ns. The error bars represent the standard deviations. The water-mediated interfacial connectivity increased throughout the binding pathway. It shows a clear anti-correlation with the RMSD of −0.75. ( d ) Examples of the pairwise water-mediated connectivity. Four different pairs are shown with known high cooperative energy. The water-mediated connectivity is formed before specific contacts are established. The connectivity values were averaged over intervals of 1 ns. Full size image Close analysis of the hydrogen-bonded water hydration shells (up to two shells for each protein) showed that the binding process started by the fusion of the hydrogen-bonded water shells (the blue-colored water in Fig. 1a ). Early on, tight water bridges form that make indirect contacts between the interfaces before the direct contacts are established ( Fig. 2b ). This shaking hands behaviour indicates an important adaptation of the water structure in the interfacial gap during the binding. We will now show how this microscopic behaviour is directly related to the water mediation and how it affects the macroscopic physical dielectric property of water. Water can mediate the interactions between two proteins with water bridges of different lengths and strengths. To account for the importance of water mediation, we introduce here a new way of characterizing the connectivity between the interfaces by means of the hydrogen-bond network, using the concept of maximum flow from mathematical graph theory [24] . This flow is a scalar measure for the connectivity between any two nodes in a network with weighted edges, taking into account their possible pathways and their weights. To study the water mediation between the interfaces, we defined a hydrogen-bonding network, using as nodes all hydrogen bond-donating and -accepting atoms at the interfaces and the water molecules in the interfacial gap (up to 0.5 nm distances from both interfaces). The hydrogen bonds were interpreted as edges connecting the nodes with their explicit energy as weights. In this way, the flow between the interfaces corresponds to the magnitude of the water-mediated connectivity. Interestingly, the total interfacial water-mediated connectivity was found to have significant values from the early stages of the transient encounter even before specific interactions are formed ( Fig. 2c ). From that it increased about twofold to threefold during the encounter complex states, especially during the first 100 ns when the rearrangement of the interfacial water molecules improved their role in mediating the binding of the interfaces. Control simulations showed that the interfacial water-mediated connectivity originates mainly from the hydrophilic and charged residues at the interfaces because mutating these residues to more hydrophobic residues abolished most of the interfacial water connectivity (see Supplementary Note 1 and Supplementary Fig. S5 ). A detailed analysis of the pairwise water mediation between all possible pairs of interfacial residues showed that most amino-acid pairs that form tight, specific interactions in the crystal complex have significant values of the water-mediated connectivity between them already in the early stages of binding before they form direct interactions (examples are presented in Fig. 2d ). This emphasizes the role of water bridges in guiding the formation of specific interactions and complements the direct interactions of those residues. The water-mediated connectivity stays significant until the stereospecific complex. Interestingly, some pairs showed experimentally measured cooperative interactions even when they are separated by distances of 0.4–1.5 nm in the bound state [14] . The cooperative nature of such weak long-range interactions (see Supplementary Table S2 ) is one of the most tantalizing issues in protein–protein interaction. This type of interactions cannot simply be explained by long-range electrostatic interactions because many non-charged residues are involved as well. We find statistically significant water-mediated connectivities for these pairs during the intermediate states and in the stereospecific complex ( Supplementary Fig. S6 ). This new finding appears to be a very plausible model to explain such indirect physical interactions. Dielectric permittivity of the water in the interfacial gap The above analysis focused on the active role of water in bridging indirect interactions that is observed in the advanced stages of binding when the interfaces are very close to each other. Now, we turn to the physical properties of the interfacial water in the early stages during the diffusive phase. The traditional continuum dielectric picture of water as a solvent suggests that the high dielectric constant of water strongly reduces the magnitude of the electrostatic interactions. Most of the available continuum electrostatic methods assume the dielectric constant of confined water or water near interfaces to be bulk-like. However, one may expect that the hydrogen-bonding network between the two proteins will affect the reorientational behaviour of water and this would also affect its dielectric properties. Therefore, we analysed the dielectric properties of the water in the interfacial gap between the interfaces when the proteins were placed at different interfacial distances (0.35–5.00 nm; see Methods ). For each distance point, the value of the dielectric permittivity was calculated from four MD simulations of 10-ns length performed with position-restrained protein backbone atoms (see Methods ). 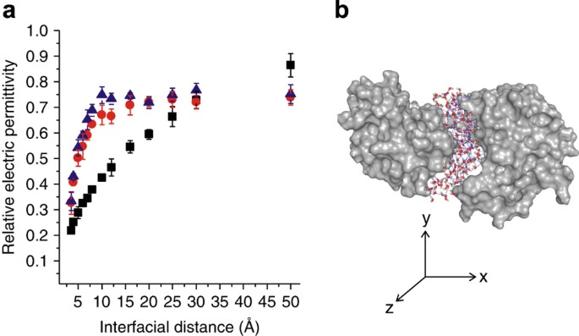Figure 3: Dielectric permittivity of the water in the interfacial gap. (a) The local dielectric behaviour in the interfacial gaps relative to the value for bulk water. The permittivity was calculated for the perpendicular direction (along thexaxis; black squares) and for the two parallel directions (red circles for theyaxis and blue triangles for thezaxis). The permittivity of the bulk water modelled by TIP4P water model56is 53±2. The values reported are taken as averages from the four simulations for every distance point and the error bars represent the standard deviation. (b) Representation of the defined interfacial gap. The interfacial gap was defined as the point within 'the displacement distance'dfrom both interfaces and not more than 1.5 nm from the line connecting the centres of geometry of the interfaces. Figure 3a (the black symbols) shows the relative perpendicular (to the interfaces) electric permittivity for each interfacial distance that was computed relative to the value of bulk water. Interestingly, the water between the two hydrophilic protein surfaces showed a strongly decreased dielectric permittivity that extended beyond 3 nm of interfacial distances. Its value is <50% of the bulk value for interfacial distances closer than 1.2 nm. Interestingly, our calculations showed that the dielectric properties of water in the interfacial gap are strongly anisotropic. A comparison of the perpendicular and the two parallel permittivities ( y and z directions) showed that the perpendicular permittivity decreases more strongly than that along the parallel directions up to distances of 3 nm. This means that water generates a preferred directionality for electrostatic interactions in the perpendicular direction that drives the interfaces towards each other (association) rather than in the parallel direction. Figure 3: Dielectric permittivity of the water in the interfacial gap. ( a ) The local dielectric behaviour in the interfacial gaps relative to the value for bulk water. The permittivity was calculated for the perpendicular direction (along the x axis; black squares) and for the two parallel directions (red circles for the y axis and blue triangles for the z axis). The permittivity of the bulk water modelled by TIP4P water model [56] is 53±2. The values reported are taken as averages from the four simulations for every distance point and the error bars represent the standard deviation. ( b ) Representation of the defined interfacial gap. The interfacial gap was defined as the point within 'the displacement distance' d from both interfaces and not more than 1.5 nm from the line connecting the centres of geometry of the interfaces. Full size image The observations of this study draw the picture of interfacial water functioning as a molecular glue sticking together the hydrophilic interfaces. In analogy to the well-known hydrophobic effect [25] , we will use the term 'hydrophilic effect' to describe the multiple roles of water in the binding of hydrophilic interfaces. Our analysis shows that the hydrophilic effect contributes to the binding of hydrophilic interfaces in two favourable ways. The first is a direct energetic contribution through the water mediation between the interfaces that stabilizes the intermediate encounter complexes before the formation of the specific direct contacts and the last specific complex. The second is indirect through the reduced dielectric properties and their directionality that is very important during the diffusive phase of binding, which is dominated by the electrostatic attraction [17] . It is a striking finding that the dielectric constant of the water in between the two reacting proteins is still significantly lower than the bulk value up to distances of a few nanometres. This strongly enhances the magnitude of the electrostatic interactions during the diffusive phase of binding. Our finding is consistent with atomic force microscopy measurement of the dielectric constant profile perpendicular to a mica surface that revealed a very long-ranged decrease even up to 10 nm from the surface [26] . We note that the computed permittivity did not converge to the value of the bulk water even at 5-nm separation. This can be partially explained by the existence of several shells of water molecules around the individual proteins, which contribute with a low permittivity to the apparent average value of the permittivity in the interfacial gap. Moreover, at large distance separation, the interfacial gap has a more inhomogeneous dielectric permittivity, which may have affected the computed value of the apparent permittivity. The stronger reduction in the perpendicular relative to the parallel directions found here also suggests an important effect of electrostatic focusing on shaping the binding funnel of the free energy landscape for association. The anisotropy of the dielectric properties observed here introduces a new complexity to the continuum treatment of water. We also demonstrated a pronounced role of the water-mediation network from the early intermediate encounter complexes. Our analysis showed that the water mediation increases continuously during the transition from the early intermediate complex to the final specific complex and thus provides a thermodynamic gradient towards the stereospecific complex as well. Such a role of bridging water molecules was proposed by Ben-Naim [27] , [28] in an early thermodynamic model for the favourable contribution of bridging water between hydrophilic molecules to free energy changes. The fingerprints of this role are reflected in the crystal structure of the complex, in which the positions of 51 water molecules were identified within 0.5 nm of both interfaces [13] (see Supplementary Figs S7 and S8 ). Nine of these water molecules have relatively low B-factors and are as ordered as protein residues at the interface with the possibility to mediate Barnase–Barstar hydrogen bonds [13] . We propose that the observed mechanism of binding is also relevant for other systems as it is very common for interfaces to be stabilized by bridging water molecules [29] , [30] , [31] , [32] , [33] . A statistical analysis of a large data set of protein complexes showed that water-mediated polar interactions are as abundant at the interfaces as direct protein–protein hydrogen bonds, [33] with an average of 15 water molecules per 1,000 Å 2 of interface area. The wet nature of hydrophilic interfaces favourably contributes to protein association in reducing the expensive desolvation penalty that would occur upon binding in the case of dry electrostatic interactions. Dry electrostatic interactions were previously shown to be unfavourable in many studies in which salt bridges buried in the protein interior were reported to be destabilizing [34] . Even simple hydrophobic interactions provided more stabilizing energy than the buried salt bridge [34] . This study shows how hydrophilic interfaces may change the physical behaviour of water from an isotropic solvent with high dielectric to an adhesive medium with reduced and directional dielectric properties. When nature wants hydrophilic interfaces to bind, bridging water is apparently an essential ingredient. MD simulation of the binding process The starting structure of the simulations was extracted from a crystal structure of a complex of Barnase–Barstar [13] (Protein Data Bank code 1BRS). Nine independent unbiased atomistic MD simulations in explicit solvent were started from different unbound conformations. These were generated by increasing the interfacial distance by 1.2–2.3 nm (see Supplementary Fig. S2 and Supplementary Table S1 ) and rotating Barstar around the line connecting the centres of masses in some cases. The five simulations that came close to the crystal structure were extended over hundreds of nanoseconds, whereas those simulations that did not come close to the crystal structure were stopped within the first 100 ns. The total length of the simulations is 1.64 μs. The OPLSAA force field [35] was used for the proteins and the TIP4P water model [36] was used for the explicit solvent. The systems were solvated in a rectangular box large enough so that the water extended at least 1.5 nm from the protein surface resulting in box dimensions of (10.2–12.3 nm)×(6.9–7.2 nm)×(6.1–6.3 nm). Four sodium counter-ions were added to make the system electrically neutral. All simulations were run with the GROMACS3.3.1 simulation package [37] . Equilibration consisted of 500 steps of steepest-descent energy minimization and a 100-ps MD simulation with harmonic position restraints using a force constant of 1,000 kJ mol −1 nm −2 for the heavy atoms in the proteins for each system. This was followed by unrestrained MD simulations in the NPT ensemble (1 atm and 310 K). For this, the system was coupled to a Berendsen external temperature bath, [38] using coupling times of 0.1 ps −1 for proteins and solvent, and the pressure was maintained constant as well by a weak coupling to a Berendsen pressure bath, [38] using a coupling time of 1 ps −1 . Long-range electrostatic interactions were computed by the particle-mesh Ewald method, [39] using Fourier spacing of 0.12 nm. Van der Waals interactions and short-range electrostatic interactions were computed within a 1.2-nm cutoff. A time step of 2.0 fs was used. Interfacial water mediation To study the role of water in bridging the interfaces and the possible change in the structure of the interfacial water, we applied the concept of network maximum flow as an index for water-mediated interfacial connectivity [24] . The hydrogen-bond network was constructed as an undirected graph, using as nodes all the hydrogen-bond donors and acceptors in the interfaces and the oxygen atoms of interfacial gap water. The water–water and water–interface hydrogen bonds were used as edges. As weights, we used the explicit hydrogen-bond energy calculated according to the explicit hydrogen-bond term from the program XPLOR [40] . Similar results were obtained with the explicit hydrogen-bonding energy term in the Grid force field [41] (see Supplementary Fig. S9 ). The flow between the interfaces was calculated after inserting a virtual super node for each interface and connecting all the nodes of the corresponding interface to this node and giving these edges infinite weights. The calculations were performed using the R package Igraph [42] . Dielectric permittivity of the water in the interfacial gap We analysed the dielectric properties of the water in the gap between the interfaces for different interfacial distances (0.35–5.0 nm). The effective local dielectric properties were characterized by using an analogue of the Kirkwood–Fröhlich formula. We show below how this formula can be applied to our anisotropic sample. This formula can also be used for the calculation of the dielectric permittivity upon application of a weak external field. Thus, we performed four different MD simulations for each interfacial distance point with two different symmetric external fields (−0.1 and 0.1 V nm −1 ), once in the direction perpendicular to the interfaces (the x axis) and once in the parallel direction (the y axis). The vector connecting the centres of geometry of the interfaces was oriented along the x axis. These electric fields are much weaker than required for saturating behaviour [43] . The permittivities reported for every distance point are average values from four simulations. The simulations were performed with the same parameters as in the binding simulations, except for additional harmonic position restraints applied to the backbone atoms of the proteins to maintain the interfacial distance. Each simulation was performed for 10 ns. The snapshots for analysis were collected every 0.25 ps from the simulation interval 2–10 ns. The interfacial gap was defined as the volume within 'the displacement distance' d from both interfaces and not more than 1.5 nm from the line connecting the centres of geometry of the interfaces. A water molecule was considered to be present in the gap if its oxygen atom was inside the gap. Formula for calculating the dielectric permittivity The macroscopic dielectric permittivity ɛ of a sample of matter is generally defined by the constitutive electrostatic relation between the local polarization P and the local macroscopic electric field [44] (Maxwell field) E . Here, ɛ and χ e are the dielectric permittivity and the electric susceptibility. In isotropic samples, ɛ and χ e are scalar quantities, whereas in non-isotropic samples, they are tensors. The macroscopic electric field E is defined as the average of the local microscopic electric field over the volume elements of the sample [45] , [46] , [47] , [48] . In general, the polarization P also has terms in higher powers of E . Yet, the constitutive relation considers only the linear term. Thus, we can write Equation (1) in the following way: To simplify the notation, we used the vectorial components in the direction of a unit vector e without loss of generality. M is the total dipole moment of the sample P·e =〈 M·e 〉/ V and V is the volume of the considered sample. The dielectric constant of a polar liquid was found to be related to the molecular dipole moment [49] and to the fluctuations of the total dipole moment for a spherical sample of liquid in the Kirkwood–Fröhlich relation [50] , [51] . Similar approaches were applied to computer simulations of isotropic polar liquids [52] , [53] for the entire system. However, our sample volume, the interfacial gap between the two proteins, is anisotropic and has a non-standard shape so that the derivation of the fluctuation formula has to be adapted to this case. The following derivation follows the summary of Böttcher [54] . The macroscopic electric field at the volume occupied by a molecule is the superposition of the field generated by all other molecules ('the internal field E i ') and the field generated by the molecule itself [54] . Onsager showed that only a part of the internal field influences the orientation of the dipoles in the electrical field, which was called as the directing field E d by Böttcher [54] . The rest of the internal field was termed the Onsager reaction field [49] R . This reaction field is generated by the surrounding as a response to the field of the molecular dipole of the molecule. Interestingly, this reaction field is oriented always parallel to the dipole of the molecule and thus does not affect its orientation. We now rewrite Equation (2) by expanding the variable of the partial derivative: For an infinite sample of isotropic liquid, the directing field equals the externally applied field. As this is not the case in general, we used in Equation 3 the directing field E d instead of E 0 (which was used in the case of isotropic sample [54] ) and followed the derivation of King and Warshel [46] (see Equation 14 in reference 46 ): The notation 〈 〉 Ed means that the averages are taken for the given value of E d . For a sample of non-polarizable spherical molecules carrying only a permanent dipole, the directing field E d equals the field in the cavity (cavity field E c ) when the molecules of the sample are removed and the surrounding molecules are relaxed to remove their interactions with the dipoles [54] (the reaction field R ; see Böttcher [54] p.174). The cavity field in a spherical cavity inside a dielectric medium of dielectric ɛ s generated as a response to a homogenous externally applied field is known to be uniform and given through the relation [53] : On the other hand, the field in a dielectric sphere of permittivity ɛ inside a dielectric medium of permittivity ɛ s is related to the externally applied field E 0 through the relation [54] : Comparing Equations (5) and (6) gives the relation between E and E d for a spherical sample shape: To find the relation between E d and the macroscopic field E in our sample volume (the interfacial gap), we followed the assumption of Onsager [49] that the entire liquid volume is occupied by the solvent molecules. Taking into account that the TIP4P water molecules have spherical shape, we can consider every water molecule in the sample as a probe of the dielectric constant of the sample volume ɛ . We will assume that every water molecule is surrounded by the sample volume ɛ s =ɛ . This assumption is well justified as most of the water molecules are in the sample volume. Moreover, the value of ɛ s has a small influence on the calculated ɛ if ɛ s has a value close to ɛ . Under this assumption, the derivative ∂ ( E d ·e )/ ∂E·e for all the molecules in the sample will be homogenous. With ɛ s = ɛ and from Equation (7) we obtain: Substituting Equations (8) and (4) in Equations (3) yields: This equation is an analogue of the Kirkwood–Fröhlich fluctuation formula for one direction and was derived by King and Warshel [46] for a spherical sample to calculate the dielectric constant inside the protein. It can also be used when external fields are applied. How to cite this article: Ahmad, M. et al . Adhesive water networks facilitate binding of protein interfaces. Nat. Commun. 2:261 doi: 10.1038/ncomms1258 (2011).